SharedVH1-46gene usage by pemphigus vulgaris autoantibodies indicates common humoral immune responses among patients Pemphigus vulgaris (PV) is a potentially fatal blistering disease caused by autoantibodies (autoAbs) against desmoglein 3 (Dsg3). Here, we clone anti-Dsg3 antibodies (Abs) from four PV patients and identify pathogenic VH1-46 autoAbs from all four patients. Unexpectedly, VH1-46 autoAbs had relatively few replacement mutations. We reverted antibody somatic mutations to their germline sequences to determine the requirement of mutations for autoreactivity. Three of five VH1-46 germline-reverted Abs maintain Dsg3 binding, compared with zero of five non-VH1-46 germline-reverted Abs. Site-directed mutagenesis of VH1-46 Abs demonstrates that acidic amino-acid residues introduced by somatic mutation or heavy chain VDJ recombination are necessary and sufficient for Dsg3 binding. Our data suggest that VH1-46 autoantibody gene usage is commonly found in PV because VH1-46 Abs require few to no mutations to acquire Dsg3 autoreactivity, which may favour their early selection. Common VH gene usage indicates common humoral immune responses, even among unrelated patients. Pemphigus vulgaris (PV) is a prototypic autoimmune disease in which autoantibodies (autoAbs) to the keratinocyte cell adhesion molecule desmoglein (Dsg) 3 can cause potentially fatal blistering of the skin and mucous membranes. The pathogenicity of anti-desmoglein 3 (Dsg3) antibodies (Abs) in PV has been experimentally validated, indicating that Dsg3 autoAbs are necessary and sufficient (even in the absence of complement or immunoglobulin G (IgG) Fc) to cause characteristic suprabasal skin blisters in passive transfer models [1] , [2] , [3] , [4] . The clinical and histologic sites of blister formation in PV are concordant with the expression pattern of Dsg isoforms and the autoAb profile in patients’ sera. Dsg3 is predominantly expressed in the basal keratinocytes of the skin and basal and suprabasal keratinocytes of the mucous membranes, whereas Dsg1 is expressed in an inverse pattern, with highest expression levels in the superficial epidermis and low level or no expression in the basal keratinocytes of the skin or mucous membranes, respectively [5] , [6] . Almost all patients with mucosal-dominant PV demonstrate Dsg3 autoAbs, and patients with mucocutaneous PV have autoAbs targeting both Dsg3 and Dsg1 (refs 7 , 8 ). The lack of skin blistering in mucosal-dominant PV is attributed to compensatory adhesion by Dsg1, which is expressed in the basal keratinocytes of the skin but not the mucosa [5] , [9] . Epitope mapping studies have shown that pathogenic autoAbs preferentially target calcium-sensitive conformational epitopes in the Dsg extracellular (EC) 1–2 domains [1] , [10] , where residues important in the trans- and cis-adhesive interactions of the Dsgs are thought to reside [11] , [12] . One of the fundamental questions in PV, as in all autoAb-mediated diseases, is how autoreactive Abs arise. Several studies have investigated the origins of autoreactive T cells in PV. The human leukocyte antigen (HLA) locus is the strongest genetic determinant of PV susceptibility in genome-wide association studies [13] , with specific associations to HLA-DQB1*0503 and HLA-DRB1*0402 alleles [14] , [15] . Interestingly, similar low frequencies of Dsg3-autoreactive T cells are observed in PV patients and HLA-matched unaffected individuals [16] . However, CD4 + CD25 + autoreactive T cells secreting IL-10 were identified in 17% of PV patients compared with 80% of HLA-matched unaffected controls, suggesting that T regulatory cell subsets may be important for the maintenance of tolerance in unaffected carriers of PV susceptibility alleles [17] . We and others have characterized anti-Dsg3 B-cell repertoires from PV patients to better understand the genetic diversity, clonal lineages and functional significance of autoreactive B cells in PV [10] , [18] , [19] . We hypothesize that shared antibody variable region gene usage and/or amino-acid sequences would be observed in PV autoAbs, since only a limited number of variable region genes would be expected to encode Abs capable of binding to pathogenic amino-terminal epitopes of Dsg3. We find that VH1-46 anti-Dsg3 Ab gene usage is shared across PV patients, which we propose may occur because VH1-46 anti-Dsg3 Abs are Dsg3-reactive when unmutated or require very few somatic mutations to acquire Dsg3 autoreactivity. 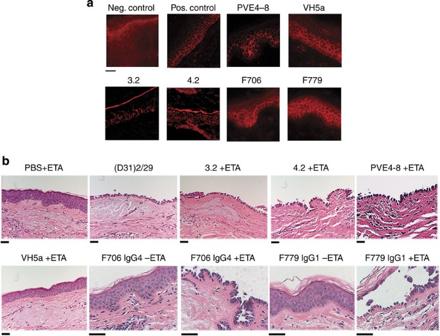Figure 1: Anti-Dsg3 mAbs reproduce the PV phenotype. (a) Indirect IF staining of human skin with scFv mAbs demonstrates cell surface binding typical of PV. Negative control is an scFv mAb against an irrelevant Ag. Positive control is a previously characterized anti-Dsg3 scFv mAb, (D31)2/2918. Scale bar, 20 μM. (b) VH1-46 mAbs, but not VH5a mAb, induce suprabasal skin blisters in human skin organ culture. Scale bar, 100 μM. Data are representative of three independent experiments. Human monoclonal Dsg3 Abs reproduce the PV phenotype We cloned anti-Dsg3 monoclonal Abs (mAbs) from the peripheral blood of four patients with active untreated PV ( Table 1 ), using the techniques of antibody phage display (patients 1–2) and heterohybridoma (patients 3–4), as described in Methods. The characterization of mAbs from patient 1, including epitope characterization, immunofluorescence (IF) staining, pathogenicity and antibody gene usage was in part previously reported [18] . Using EDTA instead of acid elution during phage library panning to enrich for mAbs binding calcium-sensitive epitopes, we identified anti-Dsg3 mAbs using one additional heavy chain, for a total of 16 unique heavy chains representing six CDR3 families (clonal lineages) from patient 1. In patient 2, we identified three unique heavy chains representing three CDR3 families. We identified one unique antibody from each of patients 3 and 4. The mAb from patient 3 has previously been reported as PVMAB786 (ref. 20 ). Table 1 Genetic and functional characteristics of anti-Dsg3 mAbs isolated from four PV patients. Full size table Across all four patients, we identified a total of 21 unique heavy chains representing 11 B-cell clonal lineages, defined by the heavy chain CDR3 sequence ( Table 1 and Supplementary Table 1 ). Eight clonal lineages bound Dsg3 only, and three clonal lineages bound both Dsg3 and Dsg1. The binding pattern to Dsg isoforms was the same within each CDR3 clonal lineage, indicating that the differences in somatic mutations observed in these clonal lineages did not affect Dsg isoform specificity. Most mAbs bound to calcium-sensitive epitopes, as determined by greater than 50% inhibition of Dsg3 enzyme-linked immunosorbent assay (ELISA) binding by EDTA ( Table 1 ). 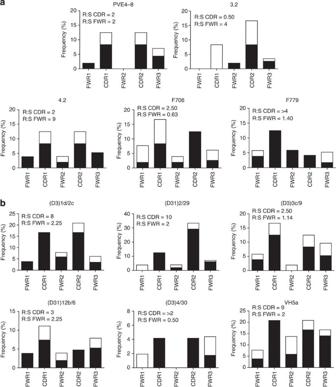Figure 2: VH1-46 anti-Dsg3 mAbs have relatively few CDR replacement mutations. Frequency of replacement (R, black) and silent (S, white) mutations in the CDRs and FWRs are shown for (a) VH1-46 anti-Dsg3 mAbs and (b) select members of other anti-Dsg3 clonal lineages. ‘>N’=N/0. VH1-46 Abs have relatively low R:S ratios in the CDRs compared with the FWRs, represented by the proportion of the bar that is black. In contrast, VH1-69 anti-Dsg mAbs ((D31)2/29 and (D3)1d/2c), have more frequent R mutations and elevated R:S ratios in the CDRs compared with the FWRs, with statistical evidence of positive antigen-driven selection (shown inSupplementary Table 3). We further determined the Dsg3 EC domain specificity of each mAb by immunoprecipitation of chimeric Dsg domain-swapped molecules ( Table 2 ). Most mAbs bound the EC1 domain of Dsg3, but three single-chain variable fragment (scFv) mAbs from patients 1 and 2 (PVE4-8, 3.2, 4.2) recognized EC1 and 3. The cross-reactivity with EC1 and EC3 was dependent on the heavy chain, as a mAb using the identical 3.2 heavy chain paired with a different light chain also recognized EC1 and 3 ( Supplementary Table 2 ). Polyclonal serum IgG from the patient from whom we cloned the mAbs recognized similar Dsg3 EC domains as the mAbs isolated from that patient. Table 2 Epitope mapping of PV serum IgG and the PV mAbs isolated from each patient against Dsg3 EC domains. Full size table Binding of mAbs to the surface of human keratinocytes was confirmed by indirect IF staining of normal human skin sections ( Fig. 1a ), similar to indirect IF patterns typical of PV sera. All five VH1-46 anti-Dsg3 mAbs, in the presence of exfoliative toxin to inactivate compensatory adhesion by Dsg1, induced suprabasal blisters in human skin explants ( Fig. 1b ). The VH5a anti-Dsg3 mAb did not cause epidermal blisters despite detectable binding to the cell surface of human keratinocytes by direct IF analysis. Figure 1: Anti-Dsg3 mAbs reproduce the PV phenotype. ( a ) Indirect IF staining of human skin with scFv mAbs demonstrates cell surface binding typical of PV. Negative control is an scFv mAb against an irrelevant Ag. Positive control is a previously characterized anti-Dsg3 scFv mAb, (D31)2/29 [18] . Scale bar, 20 μM. ( b ) VH1-46 mAbs, but not VH5a mAb, induce suprabasal skin blisters in human skin organ culture. Scale bar, 100 μM. Data are representative of three independent experiments. Full size image Collectively, these data indicate that the anti-Dsg3 mAbs that we have isolated reproduce the immunochemical and functional characteristics of PV serum IgG. VH1-46 gene usage is shared among PV patients Analysis of variable region gene usage revealed that mAbs using VH1-46 were identified in all four patients ( Table 1 ), including one patient with two clonally unrelated VH1-46 mAbs (patient 2). VK2-24 light chain gene usage was shared in two VH1-46 heterohybridoma mAbs isolated from patients 3 and 4, but no VK/VL gene usage was found in common among all four patients. Patient 1 additionally demonstrated three clonally expanded families using VH1-69 (seven unique members), VH3-07 (three unique members) and VH4-04 (three unique members). All mAbs had higher frequencies of mutations in their complementarity determining regions (CDRs) compared with the framework regions (FWRs) ( Fig. 2 ). This pattern is typical of somatically mutated (SM) antibody sequences due to the uneven distribution of somatic mutation hot and cold spots among the CDRs and FWRs and suggests that the mutations are physiologic rather than errors during PCR amplification, which would result in similar frequencies of mutations across the antibody sequence. 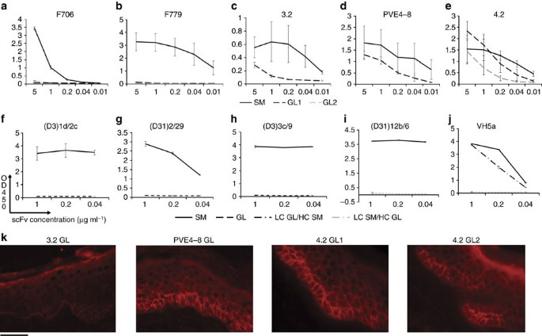Figure 3: VH1-46 mAbs require few to no somatic mutations to bind Dsg3. (a) F706 germline-reverted (GL) and (b) F779GL Abs do not bind Dsg3. (c) 3.2 GL Ab binds Dsg3 by ELISA with reduced affinity (specificity of binding confirmed by surface plasmon resonance,Table 3). (d) PVE4-8 GL and (e) 4.2 GL Abs retain binding to Dsg3 by ELISA. Black/grey hatched lines indicate GL1/2 Abs, respectively. (f–j) Germline-reverted non-VH1-46 mAbs do not demonstrate binding to Dsg3 by ELISA. GL LC/HC recombinant Abs were generated for those mAbs that were insoluble in their fully GL state. (k) Indirect IF (IIF) staining of human skin confirms Dsg3 autoreactivity of PVE4-8 GL and 4.2 GL Abs in native skin tissue. IIF binding of 3.2 GL was not detectable, presumably due to low affinity. Scale bar, 20 μM. Error bars indicate s.e.m. Data are representative of three to five independent experiments. Interestingly, VH1-46 mAbs had a relatively low number of replacement mutations in the CDRs (median 4, range 2–5) compared with non-VH1-46 mAbs (median 8, range 2–10) ( P ≤0.01 by Wilcoxon rank-sum test) ( Supplementary Table 3 ). Correspondingly, many VH1-46 mAbs had low replacement to silent (R:S) mutation ratios in the CDRs relative to the FWRs, with CDR values >2.9 typically being observed in Abs that have undergone positive antigen-driven selection [21] ( Fig. 2a ). Statistical analysis of somatic mutations using a Bayesian estimation (BASELINe) test [22] , [23] , which compares the observed versus expected frequency of replacement mutations under the null hypothesis of no selection, indicated that VH1-46 mAbs did not demonstrate statistically significant evidence of positive antigen-driven selection in the CDRs ( Supplementary Table 3 ). In contrast, VH1-69 clonal lineage 1 demonstrated statistically significant evidence of positive antigen-driven selection in the CDRs. In addition, several members in VH1-69 clonal lineage 2 showed a trend towards positive antigen-driven selection (0.05< P <0.1 highlighted in light grey), with increasing sigma values reflecting increasing selection pressures among members of the lineage. Figure 2: VH1-46 anti-Dsg3 mAbs have relatively few CDR replacement mutations. Frequency of replacement (R, black) and silent (S, white) mutations in the CDRs and FWRs are shown for ( a ) VH1-46 anti-Dsg3 mAbs and ( b ) select members of other anti-Dsg3 clonal lineages. ‘>N’=N/0. VH1-46 Abs have relatively low R:S ratios in the CDRs compared with the FWRs, represented by the proportion of the bar that is black. In contrast, VH1-69 anti-Dsg mAbs ((D31)2/29 and (D3)1d/2c), have more frequent R mutations and elevated R:S ratios in the CDRs compared with the FWRs, with statistical evidence of positive antigen-driven selection (shown in Supplementary Table 3 ). Full size image VH1-46 mAbs require few to no mutations to bind Dsg3 The relative paucity of replacement mutations in the CDRs of VH1-46 mAbs and the lack of evidence of positive selection for those mutations prompted us to investigate whether the VH1-46 mAbs identified from PV patients required somatic mutations to bind Dsg3. We reverted SM residues in the V(D)J gene segments to their corresponding germline (GL) sequences and tested for their ability to bind Dsg3 by ELISA and indirect IF staining of human skin. Germline predictions were identified by analysis of variable regions with three sequence alignment programs, SODA, Vbase2 and IMGT/V-QUEST. Some mAbs had more than one GL sequence prediction due to different D gene assignments, and hence multiple GL versions were evaluated ( Supplementary Table 1 ). F706GL and F779GL1/GL2 mAbs were unable to bind Dsg3 in the absence of somatic mutations ( Fig. 3a,b ). 3.2 GL demonstrated weak binding to Dsg3 by ELISA ( Fig. 3c ), with no detectable IF staining of human skin ( Fig. 3k ). PVE4-8GL and 4.2GL1/GL2 maintained binding to Dsg3 by ELISA ( Fig. 3d,e ), confirmed by indirect IF staining of human skin ( Fig. 3k ). None of the VH1-46 SM/GL mAbs were polyreactive, as measured by Hep2 IF and ELISA ( Supplementary Fig. 1 ). We also reverted somatic mutations in non-VH1-46 anti-Dsg3 mAbs. (D3)4/30GL ( VH3-30 ) was insoluble and was unable to be tested. (D3)1d/2c ( VH1-69 ), (D31)2/29 ( VH1-69 ), (D31)3c/9 ( VH3-07 ), (D31)12b/6 ( VH4-04 ) and VH5a ( VH5a ) all required somatic mutations to bind Dsg3 ( Fig. 3f–j ). Mutation reversion in only the light chain or only the heavy chain indicated that the heavy chain is more important for determining binding to Dsg3, as indicated for F706, F779, (D31)2/29, 4.2, (D31)12b/6 and VH5a ( Fig. 3 and Supplementary Fig. 2 ). Figure 3: VH1-46 mAbs require few to no somatic mutations to bind Dsg3. ( a ) F706 germline-reverted (GL) and ( b ) F779GL Abs do not bind Dsg3. ( c ) 3.2 GL Ab binds Dsg3 by ELISA with reduced affinity (specificity of binding confirmed by surface plasmon resonance, Table 3 ). ( d ) PVE4-8 GL and ( e ) 4.2 GL Abs retain binding to Dsg3 by ELISA. Black/grey hatched lines indicate GL1/2 Abs, respectively. ( f – j ) Germline-reverted non-VH1-46 mAbs do not demonstrate binding to Dsg3 by ELISA. GL LC/HC recombinant Abs were generated for those mAbs that were insoluble in their fully GL state. ( k ) Indirect IF (IIF) staining of human skin confirms Dsg3 autoreactivity of PVE4-8 GL and 4.2 GL Abs in native skin tissue. IIF binding of 3.2 GL was not detectable, presumably due to low affinity. Scale bar, 20 μM. Error bars indicate s.e.m. Data are representative of three to five independent experiments. Full size image We evaluated the kinetics and affinity of mAb binding to Dsg3 by surface plasmon resonance, using Dsg3-Fc recombinant fusion protein as ligand and scFv mAbs as soluble analyte. Most mAbs conformed to a 1:1 Langmuir binding model. Similar to their ELISA binding curves, 4.2 GL and PVE4-8GL demonstrated comparable (approximately twofold lower) binding affinities to their SM derivatives. 3.2 GL demonstrated specific association with Dsg3 with 80-fold lower affinity than 3.2SM, in agreement with the left shift in the ELISA binding curves ( Fig. 3c ). A summary of the kinetic data appears in Table 3 . Surface plasmon resonance curves are presented in Supplementary Fig. 3 . Table 3 Kinetic data of anti-Dsg3 mAbs measured by surface plasmon resonance. Full size table AK23 is a pathogenic mouse anti-Dsg3 mAb isolated from an active immune mouse model of PV [24] , [25] and is also pathogenic in human skin [26] . Interestingly, AK23 uses the murine VH1-53 gene segment, whose closest human homologue is VH1-46 ( Supplementary Fig. 4 ). AK23 also shows a low frequency of somatic mutations in the CDRs, with only one replacement mutation in the CDR2 compared with the mouse germline VH1-53 sequence, and two amino acid CDR changes from the human germline VH1-46 sequence. These data further support the potential for relatively unmutated VH1-46 Abs to bind human Dsg3. Acidic amino acids in the VH1-46 CDRs confer Dsg3 binding To identify amino-acid sequences required for Dsg3 binding, we compared the SM and GL sequences of the two Abs that lost Dsg3 binding on germline reversion to determine which mutations are necessary and sufficient to confer Dsg3 binding. Both F706SM and F779SM mAbs demonstrated identical acidic amino-acid mutations in the same position of the heavy chain CDR2 and light chain CDR1 ( Supplementary Table 1 ). To test whether these amino acids were necessary for Dsg3 binding, we mutated only these acidic residues to their polar analogues (D/E>N/Q). These two mutations abolished Dsg3 binding in F779SM D/E>N/Q ( Fig. 4a ). Conversely, to test whether these acidic amino-acid residues are sufficient to confer Dsg3 binding, we mutated just these two amino acids in the germline-reverted Abs back to the acidic amino-acid residue present in the SM version. In F779GL1, reintroduction of these two acidic amino-acid residues was sufficient to restore Dsg3 binding ( Fig. 4a ). Reintroduction of the two acidic amino-acid residues was not sufficient to restore Dsg3 binding to F779GL2, suggesting that the presence of acidic residues, in concert with other mutations in the CDR3, confer Dsg3 binding to that Ab. F706SM D/E>N/Q and F706GL+D/E were insoluble and could not be effectively produced, but reintroduction of these two acidic residues into a non-binding F706GL2 Ab that maintained the original CDR3 similarly restored Dsg3 binding ( Fig. 4b ). 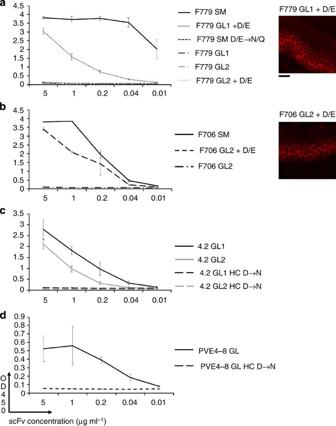Figure 4: Acidic amino-acid residues in the CDRs confer Dsg3 binding. (a) Dsg3 autoreactivity of F779SM, F779 germline-reverted (GL) in which all somatic mutations have been removed, F779SM D/E>N/Q in which only two acidic amino-acid residues in the heavy chain CDR2 and light chain CDR1 are mutated to their polar analogues, and F779GL+D/E, in which only the two acidic somatic mutations are reintroduced into the GL Ab. Binding of F779GL1+ D/E (a) and F706GL2+D/E (b) to native human skin tissue was confirmed by indirect IF. (b) Dsg3 autoreactivity of F706SM, F706GL2 and F706GL2+D/E is similar to that seen for F779. (c) 4.2GL1/GL2 both retain binding to Dsg3, but removal of two acidic residues in the heavy chain CDR3 (4.2GL1/GL2 D>N) abolished binding by ELISA. (d) PVE4-8GL retains binding to Dsg3, which depends on three acidic residues in the heavy chain CDR3 (PVE4-8 GL HC D>N). Scale bar, 20 μM. Errors bars indicate s.e.m. Data are representative of three independent experiments. Figure 4: Acidic amino-acid residues in the CDRs confer Dsg3 binding. ( a ) Dsg3 autoreactivity of F779SM, F779 germline-reverted (GL) in which all somatic mutations have been removed, F779SM D/E>N/Q in which only two acidic amino-acid residues in the heavy chain CDR2 and light chain CDR1 are mutated to their polar analogues, and F779GL+D/E, in which only the two acidic somatic mutations are reintroduced into the GL Ab. Binding of F779GL1+ D/E ( a ) and F706GL2+D/E ( b ) to native human skin tissue was confirmed by indirect IF. ( b ) Dsg3 autoreactivity of F706SM, F706GL2 and F706GL2+D/E is similar to that seen for F779. ( c ) 4.2GL1/GL2 both retain binding to Dsg3, but removal of two acidic residues in the heavy chain CDR3 (4.2GL1/GL2 D>N) abolished binding by ELISA. ( d ) PVE4-8GL retains binding to Dsg3, which depends on three acidic residues in the heavy chain CDR3 (PVE4-8 GL HC D>N). Scale bar, 20 μM. Errors bars indicate s.e.m. Data are representative of three independent experiments. Full size image For mAbs that maintained Dsg3 binding after germline reversion (4.2 and PVE4-8), we suspected that amino-acid residues in their CDR3, which were presumably introduced during V(D)J recombination, would be essential for Dsg3 binding. Sequence analysis of 4.2 and PVE4-8 indicated several acidic amino-acid residues in the heavy chain CDR3s ( Supplementary Table 1 ). To test whether these residues were necessary for Dsg3 binding, we mutated only the acidic amino-acid residues in the HC-CDR3 of 4.2GL1/GL2 and PVE4-8GL. Both 4.2GL1/GL2 ( Fig. 4c ) and PVE4-8GL ( Fig. 4d ), when stripped of acidic amino-acid residues in the heavy chain CDR3, lost the ability to bind Dsg3 by ELISA. Taken together, these data indicate that acidic amino-acid residues in the CDRs of VH1-46 mAbs are necessary and sufficient to confer binding to Dsg3. We investigated whether VH1-46 polymorphisms could introduce acidic amino-acid residues into the CDRs, which might have predisposed VH1-46 naïve B cells to Dsg3 reactivity. Thirty-five single nucleotide variants (SNVs) of VH1-46 have been previously identified in the 1000 Genomes Project ( Supplementary Table 4 ). We sequenced VH1-46 immunoglobulin M (IgM) cDNA from PV patients 1 and 2 and found that they matched the most common VH1-46 allele, designated *01. 8/35 SNVs (including the second most common allelic variant of VH1-46 with a minor allele frequency of 15.6%, designated *03) do not change the amino-acid sequence and hence would not affect antibody specificity. 19/35 SNVs encode a single amino-acid change in the FWRs, and 8/35 SNVs would change one amino acid in the CDR1-2 sequence, including one that would introduce an acidic amino-acid residue into the CDR1. However, none of these 35 SNVs were observed in PV patients 1–2, and none of the CDR1-2 amino-acid variants were observed in VH1-46 Abs from PV patients 3–4, indicating that VH1-46 polymorphisms likely did not contribute to PV susceptibility in these patients. AutoAb repertoire cloning has revealed shared VH1-46 gene usage among Dsg3 autoAbs in four PV patients, a novel finding that indicates common humoral immune responses among PV patients. Our study suggests that VH1-46 autoAb gene usage is commonly found among PV patients because VH1-46 Abs bind Dsg3 when unmutated or require very few amino-acid mutations to acquire Dsg3 reactivity, which may favour their early selection in the autoimmune response. The detection of VH1-46 anti-Dsg3 mAbs in four different PV patients using both phage display and heterohybridoma techniques makes it unlikely that the finding of VH1-46 autoAb gene usage is an artifact of any one technique and further validates the ability of phage display to identify disease-relevant clones. Phage display previously identified VH5 -51 gene usage by transglutaminase autoAbs in celiac disease patients, which was subsequently validated by single-cell PCR [27] , [28] ; several Abs cloned using the two different techniques even demonstrated the same heavy and light chain variable region gene pairings. A prior study of one paraneoplastic pemphigus patient using phage display identified VH1-46 anti-Dsg3 mAbs that induced suprabasal blisters in human skin explants [29] . Paraneoplastic pemphigus is a different disease with autoAbs to multiple antigenic targets, but nevertheless, this study supports our finding that VH1-46 is commonly used among anti-Dsg3 Abs. VH1-46 is also the closest match for the heavy chain amino-acid sequence of AK23 (ref. 25 ) ( Supplementary Fig. 4 ), a pathogenic mouse anti-Dsg3 mAb isolated from an active immune mouse model of PV [24] . One prior study also generated heterohybridoma fusions from PV patients [19] ; however, none of the isolated mAbs could bind Dsg3 endogenously expressed in human skin and thus, their biological relevance is questionable. Another study isolated 15 anti-Dsg3 mAbs from the CD22+ memory B-cell subset of two PV patients and did not find VH1-46 gene usage [10] , although one patient was on steroid therapy and their B-cell selection strategy excluded plasma cells. In contrast, our study encompassed all peripheral blood B lineage cells (through inclusion of all peripheral blood mononuclear cells or negative selection of non-B lineages) from patients who were not on systemic immunosuppressive therapy. It may also be relevant that VH1-46 anti-Dsg3 mAbs on average demonstrate an almost log-fold lower affinity for Dsg3 binding compared with the more highly mutated non-VH1-46 mAbs ( Table 3 ); for example, PVE4-8 was not identified in PV patient 1 through routine panning and was isolated by eluting with EDTA, which we expected would enrich for only pathogenic clones. In addition, VH1-46 autoAb gene usage is not commonly found in other autoimmune blistering diseases, including anti-Dsg1 mAbs from patients with pemphigus foliaceus [30] , [31] , and anti-BP180 (ref. 32 ) or anti-BP230 (ref. 33 ) mAbs from patients with bullous pemphigoid. Collectively, the data support the pathogenic relevance of VH1-46 autoAb gene usage in PV. Epitope mapping indicates that all the anti-Dsg3 mAbs identified from these four PV patients recognize Dsg3 epitopes in the EC1 domain, where amino-acid residues important in the trans- and cis-adhesive interactions of the Dsgs are located [11] , [12] . AutoAbs targeting EC1 were previously observed in 91% of PV patients [34] and were found in all four patients in this study ( Table 2 ). We identified three VH1-46 mAbs (3.2, 4.2, PVE4-8) from two different patients that also strongly reacted with Dsg3 EC3 domain. This epitope pattern was predominantly determined by the heavy chain, since these mAbs had light chains using two different VL gene segments, we also identified mAbs using the same VL gene segments that did not bind Dsg3, and furthermore, a mAb pairing the 3.2 heavy chain with a different light chain still bound the same EC1 and 3 epitopes ( Supplementary Table 2 ). Serum Abs from patient 2 recognized epitopes in EC1-4, supporting the physiologic relevance of the mAbs isolated from that patient. Serum Abs from patient 1 bound EC1 but not EC3, suggesting that the VH1-46 Ab did not comprise a significant portion of circulating serum Abs in patient 1. We suspect that the ability of these VH1-46 mAbs to cause skin blisters relies on recognition of EC1 epitopes, because adhesion domains within EC3 have not been described for Dsg3. We are currently pursuing several methods to better characterize the molecular interactions of each mAb with Dsg3. It is relevant to discuss that anti-Dsg mAbs and serum IgG have previously been distinguished as ‘pathogenic’ or ‘nonpathogenic’, the former reflecting the ability of mAbs or serum IgG fractions to cause dissociation of cultured keratinocyte cell sheets or suprabasal blisters in mouse or human skin models, and in general, correlating with recognition of Dsg3 EC1-2 domains. However, recent studies have shown that combinations of so-called ‘nonpathogenic’ anti-Dsg3 mAbs can cause pathology, which has been proposed to be due to clustering of Dsg3 on the cell surface and/or activation of cell signalling pathways [26] , [35] . Therefore, we cannot rule out a pathogenic role for EC3 domain recognition in induction or potentiation of skin blistering by these PV mAbs (for example, by allosteric inhibition, signalling, or facilitating Dsg cell surface clustering). In regard to the current study, the identification of ‘pathogenicity’, that is, the ability to cause suprabasal blisters in human skin, is important to demonstrate that the PV mAbs we have identified reproduce the PV phenotype. However, regardless of their ability to cause skin blisters in pathogenicity assays, all the anti-Dsg3 Abs we identified are ‘pathologic’, in that serum anti-Dsg3 Abs are not observed in the vast majority of non-pemphigus individuals [36] . The germline reversion studies ( Fig. 3 ) indicate that a subset of VH1-46 anti-Dsg3 mAbs retain Dsg3 binding in the absence of somatic mutations. The VH1-46 SM and germline-reverted Abs are Dsg3 reactive, but not polyreactive. Polyreactivity has been proposed to increase the apparent affinity of HIV Abs to sparse ligands such as gp120 by heteroligation of gp120 with self-antigens, thereby increasing the likelihood of B-cell activation [37] . Polyreactivity of B cells is commonly observed in patients with rheumatoid arthritis, systemic lupus erythematosus and multiple sclerosis [38] , [39] , [40] . The lack of Hep2 polyreactivity observed in PV anti-Dsg3 mAbs ( Supplementary Fig. 1 ) does not rule out polyreactivity with other human autoantigens, but is consistent with the observation that PV VH1-46 mAbs contain negatively charged amino-acid residues in their CDRs, whereas polyreactive Abs tend to have basic CDR residues that facilitate binding of negatively charged epitopes in nucleic acid and phospholipid autoantigens [41] . A previous study has shown that four anti-Dsg3 mAbs lost binding to Dsg3 on germline reversion [10] . None of these mAbs used VH1-46 . In addition, the majority of these Abs were more highly mutated, with patterns of mutation supporting positive antigen-driven selection, consistent with their memory B-cell origin. Similarly, we found that the more highly mutated non-VH1-46 anti-Dsg3 mAbs depended on somatic mutation for Dsg3 binding ( Fig. 3f–j ). As the immune response towards Dsg3 matures, high levels of somatic mutation could induce Dsg3 reactivity from a broader range of VH genes, which are hence less likely to be shared among patients. In a prior study, we reported a consensus D/E-X-X-X-W motif in the heavy chain CDR3 of pathogenic anti-Dsg3 and anti-Dsg1 mAbs isolated from PV and PF patients and a mouse model of PV [42] . Two of the five pathogenic VH1-46 anti-Dsg3 mAbs share this consensus motif ( Supplementary Table 1 ). We previously investigated requirements within this motif for Dsg binding, and found that alanine replacement of the conserved acidic amino acid did not significantly affect Dsg binding (relative affinity was the same to fourfold decreased). However, mutation of the tryptophan blocked mAb pathogenicity, and mutation of all five residues in the motif abolished Dsg binding. Subsequent studies of pathogenic PV or paraneoplastic pemphigus anti-Dsg3 mAbs did not identify shared CDR3 motifs [10] , [29] . Our current study indicates that acidic amino-acid residues throughout the heavy chain CDRs of VH1-46 PV mAbs are necessary for Dsg binding ( Fig. 4 ). Collectively, these studies suggest that acidic amino-acid residues throughout the heavy chain CDRs, not only in the CDR3, are important for Dsg3 binding, and that the PV CDR3 consensus motif occurs more commonly with, but is not required for, anti-Dsg3 mAb pathogenicity. High CDR R:S ratios were observed in two VH1-69 clonal lineages we identified ( Fig. 2b ), with statistically significant evidence of positive antigen-driven selection in VH1-69 clonal lineage 1 ( Supplementary Table 3 ). Increasing sigma values within VH1-69 clonal lineage 2 indicates increasing selection pressure on these clones, suggestive of a memory B-cell (post-germinal center) origin, although the lower number of somatic mutations in these sequences may have limited our power to detect statistically significant evidence of positive antigen-driven selection ( P =0.053–0.088). In contrast, few replacement mutations and low CDR R:S ratios were observed in VH1-46 autoAbs. Significant positive selection is not detected because these Abs require no to very few mutations to bind Dsg3. Although our study does not directly investigate the cell of origin, a plasmablast origin for PV autoAbs is supported by data from pemphigus patients treated with rituximab, who demonstrate a specific decrease in serum anti-Dsg Ab titres without significant change in the levels of serum Abs against Pneumococcus or tetanus toxoid, which are produced by long-lived plasma cells [43] , [44] . In conclusion, the finding of shared VH gene usage in PV autoAbs is significant in that it indicates that autoimmunity in PV may develop through common humoral immune pathways. A prediction of our data is that PV patients harbour naïve Dsg3-autoreactive IgM+ B cells, which may be enriched in VH1-46+ B cells that acquire acidic amino acid CDR3 residues during V(D)J recombination. Dsg3-autoreactive B cells may survive because of ignorance, since Dsg3 is not expressed centrally in the bone marrow, and its expression is restricted in the periphery to stratified squamous epithelia, such that B cells would likely not encounter sufficient Dsg3 antigen to undergo clonal deletion or become anergic. Dsg3-autoreactive T cells, in contrast, should be deleted centrally in the thymus because Dsg3 is expressed under the autoimmune regulator (AIRE) promoter [45] . Ignorant B cells therefore should not receive T cell help to mature and produce high-affinity anti-Dsg3 IgG. However, a low number of Dsg3-autoreactive T cells escape into the periphery in unaffected carriers of HLA alleles associated with PV susceptibility [16] . Thus, in the setting of the appropriate co-stimulatory signals in an HLA-susceptible host, autoimmunity may mistakenly ensue. During subsequent affinity maturation of the autoimmune response to Dsg3, higher-affinity Abs created by somatic mutation and using a broader range of VH genes also contribute to the polyclonal anti-Dsg3 IgG repertoire. This model accounts for the rarity of pemphigus, since disease depends on multiple rare events to occur, including the creation of Dsg3-autoreactive B cells by V(D)J recombination in naïve B cells and/or peripheral somatic mutation in memory B cells, escape of rare Dsg3-autoreactive T cells into the periphery in HLA-susceptible individuals and breakdown of peripheral tolerance to allow autoimmune activation to occur, likely in the setting of infection or inflammation. A recent study has shown that long-term remissions of pemphigus after CD20+ B-cell depletion with rituximab are associated with specific loss of Dsg-specific B cells [46] . Interestingly, the number of Dsg3-specific IgG+, but not IgM+, B cells significantly decreased in patients in complete remission compared with those with newly diagnosed disease. These in vivo data support our model that Dsg3-specific IgM+ B cells will constantly be created through V(D)J recombination at rare but certain frequencies. Therefore, it is not necessary or possible to eliminate these Dsg3-specific pathologic precursors from the repertoire. Instead, B-cell-depletion therapy works in pemphigus by interrupting the processes that create Dsg3-specific IgG+ B cells (through somatic mutation and/or pathologic activation of naïve Dsg3-reactive IgM+ B cells). Future studies to better define B-cell tolerance checkpoints for Dsg3, characterize B-cell subset-specific repertoires to identify the relative frequencies of VH1-46 Dsg3-reactive clones, and identify possible infectious triggers of the anti-Dsg autoimmune response will improve our understanding of the causes of human autoimmunity and the most effective treatment strategies for disease. Peripheral blood collection All four patients had active mucocutaneous PV and were off systemic therapies at the time of blood draw. Peripheral blood was collected from patients following informed consent using a protocol approved by the Institutional Review Board of the University of Pennsylvania. The diagnosis of PV was established by typical clinical presentation, histology and IF. Antibody phage display Phage display was performed as previously described [18] , with the following changes. The library from patient 1 was re-panned on Dsg3 ELISA plates (MBL International) and eluted with 5 mM EDTA instead of acid glycine to enrich for Abs binding to calcium-sensitive epitopes. The library from patient 2 was panned twice, at room temperature (yielding VH5a) and 4 °C (yielding 3.2 and 4.2), because 4 °C incubation stabilized binding of a prior pathogenic anti-Dsg1 scFv (unpublished data). A fifth PV patient, from whom VH1-46, VH5-51, and two VH1-69 anti-Dsg3 mAbs were isolated and in part previously reported [42] , was not included in this study due to a sequence irregularity identified in one of the scFv mAbs. Heterohybridoma production and screening B cells were purified from whole blood by negative selection against CD2, CD3, CD16, CD36, CD56, CD66b and glycophorin A using RosetteSep (Stem Cell Technologies). For patient 1 (PV3), 10 7 B cells were stimulated with Epstein–Barr virus for 48 h before fusion with HMMA 2.5 myeloma cells as previously described [20] . For patient 2 (PV4), 3 × 10 6 B cells were stimulated using a cocktail of inactivated Staphylococcus aureus Cowan 1 strain and IL-2 for 48 h before fusion with the HMMA 2.5 heteromyeloma cell line as previously described [47] . Cell fusion mixtures were aliquoted among six 96-well plates (576 wells) and cultured. Heterohybridoma supernatants were screened for production of total IgG, as well as Dsg3-specific IgG by ELISA. Hybridomas were screened only for IgG and not IgM to more effectively capture the antigen-driven response. Anti-Dsg3-IgG-positive wells were subsequently cloned by limiting dilution. IgG subclass was identified by ELISA as previously described [48] . Antibody subcloning, expression and purification F706 IgG4 and F779 IgG1 hybridomas were subcloned into the pComb3X vector to allow production as scFv mAbs for BIAcore and germline reversion analysis. ScFv mAbs were produced and purified as previously described [18] , [49] , with the substitution of FastBreak lysis reagent (Promega) and cobalt affinity column chromatography (Talon, Clontech) for purification. Sequence and statistical analysis Messenger RNA was isolated from F706 and F779 parental heterohybridoma cell lines for cDNA synthesis (FastTrack 2.0, Invitrogen). The human antibody heavy and light chains were amplified for sequencing using human Ig-primer sets (Novagen). The nucleotide sequences were compared with the germline sequences in the Vbase2 sequence directory ( www.vbase2.org ). DNA sequences of F706 IgG4 and F779 IgG1 were deposited to GenBank. To identify somatic mutations, sequences were compared using three analysis programs, Vbase2, IMGT/V-QUEST [50] , [51] and SoDA ( https://dulci.org/soda ) [52] . Normalized frequencies of somatic mutations were calculated by dividing the number of mutations by the total number of nucleotides per antibody region, masking primer-encoded nucleotides in FWR1/FWR4. Mutations in the CDR1, 2 and 3 were reverted, sparing the N and P nucleotides. In some cases where germline sequence predictions varied among the three analysis programs due to identification of different D genes, more than one germline scFv was produced. Sequence and statistical analysis for the presence of positive or negative selection based on comparisons of observed versus expected replacement and silent mutations was performed using the BASELINe test ( http://selection.med.yale.edu/baseline/ ) [22] , [23] . This test compares the expected replacement and silent mutations, based on hotspot analysis of somatic mutation enzyme sites in each mAb, with the observed mutations to determine whether the observed mutation frequency is different from what would be expected based on random mutation (indicating positive or negative selection). Expected mutation frequencies (which are identical within each clonal lineage based on somatic mutation hot/cold spots and nucleotide substitution bias for each germline VH gene sequence) were multiplied by the total number of observed mutations to generate the expected number of mutations, which predicts how the total number of mutations would be distributed across the CDR and FWR regions for each individual clone. P- values less than 0.05 were considered significant. The amino-acid sequence of AK23 (ref. 25 ) was queried against the Mus musculus protein database ( http://blast.ncbi.nlm.nih.gov ), which identified VH1-53 as the most closely aligned VH gene segment. The nucleotide sequence of murine VH1-53 was compared with the IMGT human Ig set to identify the closest human homologue. VH1-46 IgM transcripts in patient 1 were amplified by RT–PCR using a 5′ VH1 forward primer and 3′ HSCG-M reverse primer [53] . IgM transcripts in patient 2 were amplified using a forward leader primer 5′-GTCTTCTGCTTGCTGGCTGTAGCTC-3′ or 5′-GTCTTCTGCTTGCTGGCTGTAGCAC-3′ and an IgM CH1 reverse primer 5′-CCTGGCCGGCCTGGCCGCTGGTAAGGGTTGGGGCGG-3′. Sanger sequencing of subcloned heavy chains (patient 1) or pooled PCR products (patient 2) was performed to identify VH1-46 sequences. VH1-46 SNPs from 1092 human genomes were identified using the 1000 Genomes browser ( http://www.ncbi.nlm.nih.gov/variation/tools/1000genomes ). Antibody mutation studies To construct germline-reverted scFv, germline light chains and the germline VH1-46 gene segment were synthesized as minigenes (Integrated DNA Technologies). The light chains were amplified using primers to append a 5′ SfiI site 5′-GGGCCCAGGCGGCCGAGCTC-3′ and a 3′ scFv long linker [53] ( Supplementary Methods ). The heavy chains were amplified in a two-step process to amplify the germline VH segment with a 5′ primer to append the scFv long linker 5′-GGTGGTTCCTCTAGATCTTCCTCCTCTGGTGGCGGTGGCTCGGGCGGTGGTGGGCAGGTGCAGCTGGTGCAGTCTGG-3′ and a 3′ primer encoding the heavy chain CDR3 5′-ACGCGCACAGTAATACACGGCCGTGTC-3′, followed by amplification of the germline JH gene from a pComb3X scFv with a 5′ primer overlapping the heavy chain CDR3 5′-GACACGGCCGTGTATTACTGTGC-3′ and a 3′ primer appending an SfiI site after the hemagglutinin and 6xhistidine tags 5′-GGGCCGGCCTGGCCACTAGTGACCGATGGGCCCTTGGTGGAAGCTGAGGAGACGGTGACC-3′. The complete scFvs were subsequently ligated into the SfiI site of pComb3x. Some mutated scFv were produced by synthesizing heavy and light chains as gBlocks (Integrated DNA Technologies) that were subsequently ligated together using the Gibson Assembly cloning kit (New England BioLabs). For some mAbs, the entire scFv sequence was synthesized (Invitrogen). Point mutations in scFv were performed using the Quikchange Lightning Multi Site-Directed Mutagenesis Kit (Agilent). Immunochemical studies Dsg3 ELISA (MBL International) and direct/indirect IF on human skin was performed as described [18] . Due to inefficient production of some mAbs, some SM/GL scFv ELISAs were performed with unpurified scFv bacterial lysates. To test calcium sensitivity, ELISA wells were preincubated for 30 min with either TBS/1 mM calcium chloride or TBS/5 mM EDTA and then processed as above. Hep2 IF (Euroimmun) and ELISA (IBL) were performed according to manufacturer’s protocols. Pathogenicity assays Evaluation of mAb pathogenicity using ex vivo injection of human skin organ culture was performed as described [54] , with normal human skin provided by the Penn Skin Disease Research Center. Specimens were harvested 16–18 h after mAb injection and bisected. One half was fixed in 10% phosphate-buffered formalin (Sigma) and one half was embedded in OCT (Electron Microscopy Sciences) for frozen sections and direct IF analysis to confirm Ab binding. Epitope mapping For PV sera and IgG mAbs, epitope mapping was performed as described [34] , [55] , using chimeric Dsg domain-swapped constructs generously provided by Professor Masayuki Amagai. For scFv mAbs, baculoviral supernatants containing chimeric Dsg domain-swapped molecules were incubated with scFv mAbs followed by precipitation with anti-hemagglutinin agarose (Sigma). Surface plasmon resonance Binding of scFv mAbs to Dsg3 was measured using a BIAcoreX optical biosensor. Mouse anti-human IgG Fc mAb (Biacore) was attached to a CM5 sensor chip via standard amine coupling procedures using N-hydroxysuccinimide/N-ethyl-N′-[3-(dimethylamino) propyl]carbodiimine hydrochloride (Pierce). The chip was blocked with 1 M ethanolamine, pH 8.5 for 7 min. All assays were performed in HBS-EP buffer at 25 °C (Biacore). Baculoviral Dsg3-Fc fusion protein [2] , produced as described [56] , was captured on one flow cell; a second flow cell with mouse anti-human IgG Fc mAb but no Dsg3-Fc was used as a reference cell. Binding of scFv was measured over at least three concentrations; more dilutions were performed if the initial dilutions were not sufficient to fit the kinetic data with good χ 2 values. The bulk shift due to changes in refractive index (measured on the reference cell) was subtracted from the binding signal to correct for nonspecific signals. Surfaces were regenerated with 3 M MgCl 2 . Dsg3-Fc was reproducibly recaptured for each measurement cycle, with an average level of ~500 response units. Data were initially fit to 1:1 Langmuir binding model. Abs with significant bulk change added to the fit or χ 2 values >2 were also tested against a conformational change or heterogeneous ligand model using global analysis in the BIAevaluation 3.0 software (Biacore). Accession codes : F706 heavy and light chains=DQ003033 and DQ003034; F779 heavy and light chains=HQ338093 and HQ338094; PVE4-8 scFv=KF193430; 3.2 scFv=KF193428; 4.2 scFv=KF193429. How to cite this article : Cho, M. J. et al. Shared VH1-46 gene usage by pemphigus vulgaris autoantibodies indicates common humoral immune responses among patients. Nat. Commun. 5:4167 doi: 10.1038/ncomms5167 (2014).